A seamless three-dimensional carbon nanotube graphene hybrid material Graphene and single-walled carbon nanotubes are carbon materials that exhibit excellent electrical conductivities and large specific surface areas. Theoretical work suggested that a covalently bonded graphene/single-walled carbon nanotube hybrid material would extend those properties to three dimensions, and be useful in energy storage and nanoelectronic technologies. Here we disclose a method to bond graphene and single-walled carbon nanotubes seamlessly during the growth stage. The hybrid material exhibits a surface area >2,000 m 2 g −1 with ohmic contact from the vertically aligned single-walled carbon nanotubes to the graphene. Using aberration-corrected scanning transmission electron microscopy, we observed the covalent transformation of sp 2 carbon between the planar graphene and the single-walled carbon nanotubes at the atomic resolution level. These findings provide a new benchmark for understanding the three-dimensional graphene/single-walled carbon nanotube-conjoined materials. As low-dimensional materials, graphene [1] , [2] and single-walled carbon nanotubes (SWCNTs) [3] , [4] exhibit exceptional properties such as high carrier mobility [5] , [6] , [7] , [8] , high electrical and thermal conductivity [9] , [10] , and large specific surface area (SSA) [11] . The combination of nanotube carpets and graphene is an approach to extend those properties into three dimensions [12] , [13] , [14] . However, high-quality, single- and few-walled carbon nanotube (CNT) carpets with large SSA are usually grown on alumina, an insulator that immobilizes the catalyst particles and supports efficient growth [15] , [16] . In contrast, high-quality graphene is usually produced on metal substrates such as copper or nickel [17] , [18] , [19] , [20] . These two different growth conditions hamper attempts to covalently combine the two materials during growth. As a result, attempts to grow graphene and CNT carpet hybrid material [21] , [22] , [23] , [24] have failed to match the predicted values on SSA, electrical connection or both. Several facts explain the mismatch between the experimental results and theoretical predictions: first, the quality of graphene is not well controlled. Some researchers use reduced graphene oxide instead of chemical vapour deposition-produced graphene in their study. The reduced graphene oxide is a defect-rich material compared with the models used in the theoretical calculations [12] , [13] , [14] . This inevitably leads to materials with different properties from those based on calculations. Second, the quality of the CNTs is not ideal. Many of the best properties of the general class of compounds that comprise CNTs, such as high SSA and large aspect ratio, are based on SWCNTs, which were the properties used in the theoretical modelling [12] , [13] , [14] . However, the CNTs synthesized [21] , [22] , [23] were multi-walled CNTs with large diameters that have much lower SSA and more defects when compared with SWCNTs. Third and most important, although those reports referred to the products as graphene/CNT hybrid material, the actual connection between the CNTs and graphene was not studied. The atomic structure of the graphene–CNT junction has never been observed and it is unclear in the previously published work whether there are covalent bonds that seamlessly link the graphene and CNTs. On the basis of the properties reported, it could be that many of those CNTs are physisorbed on the graphene plane rather than conjoined by sp 2 carbon to sp 2 carbon. Here we disclose a method to prepare high-quality graphene with few-walled (one- to three-walled) CNT carpets seamlessly connected via covalent bonds. Without sacrificing their stand-alone properties, the ohmic interconnected graphene and CNT carpet hybrid can be produced in a high-surface area material that can affect, for example, high-performance supercapacitor devices. Although others [25] have superbly pioneered a related growth on bulk carbon, the graphene substrate method disclosed here permits access to investigate the atomic nature of the interface between the carbon surfaces, in this case graphene, and the nanotube carpet. The atomic scale aberration-corrected scanning transmission electron microscopic (STEM) analysis gives the detailed information of the conjugated covalent bonds in the junction region, which is in agreement with previous simulation studies. Synthesis of covalently bonded graphene and CNT carpets using a floating buffer layer To simultaneously control the diameter of CNTs while forming covalent bonds between graphene and the CNT forest, we use a sandwich structure with the catalyst layer between the graphene substrate and top buffer alumina layer. There is no barrier between the graphene and nanotube carpet in this structure, and the top alumina layer acts as a floating buffer layer, assisting the formation of small-diameter CNT carpets. The growth process is diagrammed in Fig. 1 . First, the graphene is grown on a copper foil ( Fig. 1a ) [18] , [20] , then the iron catalyst and alumina buffer layer are deposited on the graphene in series by electron beam (e-beam) evaporation ( Fig. 1c ). During the growth, the catalyst and alumina are lifted up and the CNT carpet is grown directly out of the graphene ( Fig. 1d ). This growth strategy results in seamless covalent bonds between the graphene and CNT carpet. 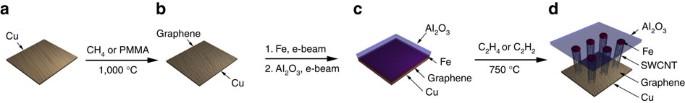Figure 1: Scheme for the synthesis of CNT carpets directly from graphene. (a) Copper foil substrate. (b) Graphene is formed on the copper foil by chemical vapour deposition (CVD) or solid carbon-source growth. (c) Iron and alumina are deposited on the graphene-covered copper foil by using e-beam evaporation. (d) A CNT carpet is directly grown from graphene surface. The iron catalyst and alumina protective layer are lifted up by the CNT carpet as it grows. Figure 1: Scheme for the synthesis of CNT carpets directly from graphene. ( a ) Copper foil substrate. ( b ) Graphene is formed on the copper foil by chemical vapour deposition (CVD) or solid carbon-source growth. ( c ) Iron and alumina are deposited on the graphene-covered copper foil by using e-beam evaporation. ( d ) A CNT carpet is directly grown from graphene surface. The iron catalyst and alumina protective layer are lifted up by the CNT carpet as it grows. Full size image Observation of the growth at the initial stage of CNT growth was sought; however, it is very fast with over 10-μm-long nanotubes grown in seconds [26] , which makes direct observation of the initial stage difficult. Alternatively, if less catalyst was used, the CNT growth can be stopped at its initial stage for direct observation due to rapid deactivation of the catalyst [27] . 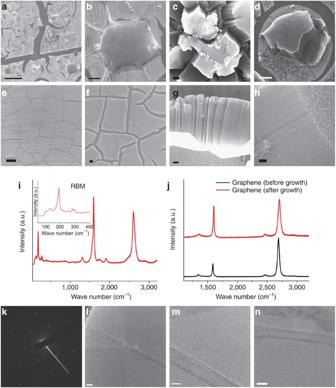Figure 2: Characterization of CNT carpet grown from graphene. (a–h) SEM images of nanotube carpet grown from a graphene-covered copper foil. (a,b) The samples grown by using 0.3 nm of iron and 3 nm of alumina. The dark regions inaare gaps in the broken alumina layer and the brighter regions are alumina-covered areas. Scale bar ina, 50 μm. (b) An enlarged image for one of the lifted areas where the CNTs were grown. Scale bar inb, 10 μm. (c,d) The samples grown by using 0.5 nm of iron and 3 nm of alumina. Scale bar incandd, 10 μm. (c) The top alumina layer is partially broken. (d) The top alumina layer is fully removed during growth. (e–h) The samples grown by using 1 nm of iron and 3 nm of alumina. (e,f) Top view of the CNT carpet on the graphene-covered copper foil. Scale bar ine, 50 μm. Scale bar inf, 10 μm. (g) The side view of the CNT carpet grown on the graphene; the height of the CNT is ~120 μm. Scale bar ing, 10 μm. (h) The close-up view on the upper portion of the CNT carpet. Scale bar inh, 1 μm. (i,j) Raman spectra of the CNT carpet and graphene. (i) Raman spectrum of the CNT carpet (excitation wavelength 633 nm). Inset: the spectrum of the radial breathing modes (RBMs). (j) Raman spectra of graphene before (black) and after (red) CNT growth (excitation wavelength 514 nm). (k) The diffraction pattern of the graphene after CNT growth. (l–n) TEM images of CNTs grown in this work. Scale bar inl,mandn, 5 nm. (l) Single-walled nanotube. (m) Double-walled nanotube. (n) Triple-walled nanotube. Figure 2a–h is the scanning electron microscope (SEM) images of samples grown using 0.3, 0.5 and 1 nm iron catalyst layers, respectively. With a 0.3-nm iron catalyst layer, the CNTs grew in isolated patches and the alumina layer was not fully lifted. With 0.5 nm of iron catalyst, although the growth was still limited to small patches, a CNT forest appeared and the alumina layer was sporadically lifted. We also observed that the top alumina layer was partially ( Fig. 2c , centre part) or fully ( Fig. 2d ) removed, which provides evidence for the alumina layer lifting mechanism. On the areas where alumina was raised ( Fig. 2c , centre part and Fig. 2d ), a bright catalyst layer was visible using SEM, indicating the tip growth ‘Odako’ (Japanese kite) mechanism [25] . When the iron catalyst layer was 1 nm thick ( Fig. 2e–h ), the CNT carpet was grown throughout the entire catalyst region and a large-scale homogeneous carpet was visible ( Fig. 2e–f ). Compared with the normal CNT carpet under super growth conditions [16] , this carpet was usually split into patches of hundreds of micrometre in size. The gaps in between were formed during the initial growth stage, when the carbon feedstock needed to pass through them to reach the catalyst. The side view of the CNT carpet in Fig. 2g shows that the CNTs can be as long as 120 μm after 10 min of growth. The carpet tip region is imaged in Fig. 2h , where the nanotubes are still well-aligned. Detailed growth optimizations are described in the Supplementary Fig. S1–S3 . Interestingly, the graphene layer was found to be essential for the CNT growth over the copper foil. Without the graphene layer, deactivation of the iron catalyst ensued ( Supplementary Fig. S2 ), presumably due to alloying. Figure 2: Characterization of CNT carpet grown from graphene. ( a – h ) SEM images of nanotube carpet grown from a graphene-covered copper foil. ( a , b ) The samples grown by using 0.3 nm of iron and 3 nm of alumina. The dark regions in a are gaps in the broken alumina layer and the brighter regions are alumina-covered areas. Scale bar in a , 50 μm. ( b ) An enlarged image for one of the lifted areas where the CNTs were grown. Scale bar in b , 10 μm. ( c , d ) The samples grown by using 0.5 nm of iron and 3 nm of alumina. Scale bar in c and d , 10 μm. ( c ) The top alumina layer is partially broken. ( d ) The top alumina layer is fully removed during growth. ( e – h ) The samples grown by using 1 nm of iron and 3 nm of alumina. ( e , f ) Top view of the CNT carpet on the graphene-covered copper foil. Scale bar in e , 50 μm. Scale bar in f , 10 μm. ( g ) The side view of the CNT carpet grown on the graphene; the height of the CNT is ~120 μm. Scale bar in g , 10 μm. ( h ) The close-up view on the upper portion of the CNT carpet. Scale bar in h , 1 μm. ( i , j ) Raman spectra of the CNT carpet and graphene. ( i ) Raman spectrum of the CNT carpet (excitation wavelength 633 nm). Inset: the spectrum of the radial breathing modes (RBMs). ( j ) Raman spectra of graphene before (black) and after (red) CNT growth (excitation wavelength 514 nm). ( k ) The diffraction pattern of the graphene after CNT growth. ( l – n ) TEM images of CNTs grown in this work. Scale bar in l , m and n , 5 nm. ( l ) Single-walled nanotube. ( m ) Double-walled nanotube. ( n ) Triple-walled nanotube. Full size image As the CNT carpet is grown directly from the graphene surface atop copper, it is difficult to observe the Raman spectrum of the graphene after growth. To solve this problem, a graphene sheet was transferred to a Si/SiO 2 wafer and the catalyst was patterned on the graphene surface using e-beam lithography. The same growth parameters that were used on the copper foil were used for the graphene on Si/SiO 2 , and the CNT carpet only grew on the area where there was a catalyst ( Supplementary Methods ). The characteristic Raman spectra of CNTs and graphene were observed from the hybrid material as shown in Fig. 2i . The G/D ratio of the CNTs is ~8:1, which is comparable to super growth CNT forests [16] . The strong radial breathing mode signals ( Fig. 2i and Supplementary Fig. S4 ) indicate the existence of high-quality small-diameter CNTs in the carpet. The graphene quality was carefully checked before and after the CNT carpet growth. The Raman spectra of graphene, before and after CNT growth, are plotted as black and red curves in Fig. 2j , respectively. There is a slight increase in both the G and D peaks after the nanotube growth. The TEM diffraction pattern ( Fig. 2k ) shows that the graphene is still monolayer after the CNT carpet growth. The increases of the G peak and D peak most likely result from a small amount of amorphous carbon deposition during growth. Additional Raman mapping experiments are shown in Supplementary Fig. S3 . The TEM images ( Fig. 2l–n ) show the typical CNTs grown under these conditions. Most CNTs in the carpet are single-walled, double-walled or triple-walled. The diameters of the CNTs are between 1 and 7 nm. The thin, top alumina layer (3 nm) is the key factor in maintaining the small diameter of the CNTs. Without the correct amount of alumina layer, the CNT diameters are usually larger than 20 nm and the carpet-like CNT forest does not form ( Supplementary Fig. S1 ). It is clear that the thin alumina layer effectively permits formation of small-diameter CNTs in the carpet even though deposited on top of the iron catalyst. High-surface area materials with efficient electrical connections and applications in supercapacitors If there are indeed C–C covalent bonds formed between the CNTs and the graphene, it should lead to efficient electrical contact between the CNT carpet and the graphene plane. To evaluate the electrical behaviour of CNT–graphene junctions, devices as seen in the SEM image in the inset of Fig. 3a were fabricated on a Si/SiO 2 wafer ( Supplementary Methods and Supplementary Fig. S5 ). The Pt and CNT carpet electrodes were fabricated on the patterned graphene. The measurements were carried out as illustrated in Fig. 3b . One micromanipulated probe tip was placed on the Pt electrode and the second tip was placed on the graphene electrode, and the I–V response was measured as curve I in Fig. 3a . The tip on the graphene electrode was then elevated, and the I–V response indicated there was no current passing through the device (curve II in Fig. 3a ). As the probe station allows relatively precise horizontal movement of the probe tip, the elevated tip was shifted horizontally to the CNT carpet electrode. Although the probe tip was still suspended above the substrate plane, it contacted the side wall of the carpet because of the height of the CNT carpet, and curve III in Fig. 3a was obtained. Curve III and curve I are almost identical, except that there is more oscillation in III, originating from the loose contact between the tip and the side wall of the nanotube carpet. This identical electrical response from CNTs or graphene to the metal electrode indicates an ohmic contact at the junction of the CNTs and graphene. Though the Ohmic contact by itself does not ensure a seamless junction, the Ohmic contact afforded is beneficial for device construction as demonstrated here. 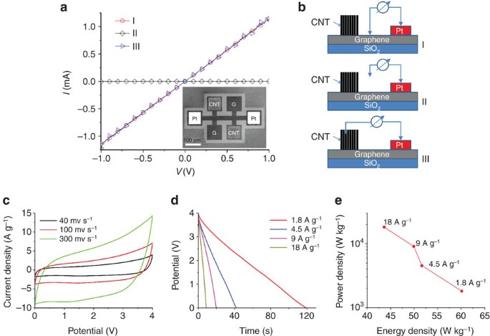Figure 3: Electrical properties of graphene and CNT carpet hybrid materials and the supercapacitor device characterization. (a–b) Characterization of the electrical properties of graphene and CNT carpet hybrid materials. (a) TheI–Vcurves of three experiments described inb. The inset is the SEM image of the device; graphene (the dark area) is patterned into a Hall-bar shape. ‘Pt’ is the platinum electrode deposited on graphene, ‘CNT’ is the CNT carpet electrode grown on graphene, ‘G’ is the bare graphene electrode. (b) Three experiments that were used to measure theI–Vresponses: I, one probe contacts the platinum electrode and the other probe on the graphene electrode; II, one probe is on the platinum electrode, the other probe is suspended above the surface; III, one probe is on the platinum electrode, the other probe is contacting the CNT carpet side walls. (c–e) Characterization of a supercapacitor made from the graphene and CNT carpet hybrid materials. (c) Cyclic voltammetry of supercapacitor device under different scan rates. (d) Galvonostatic discharge curves under different discharge currents. (e) Ragone chart of energy density versus power density; the voltage window is 4 V. Figure 3: Electrical properties of graphene and CNT carpet hybrid materials and the supercapacitor device characterization. ( a – b ) Characterization of the electrical properties of graphene and CNT carpet hybrid materials. ( a ) The I–V curves of three experiments described in b . The inset is the SEM image of the device; graphene (the dark area) is patterned into a Hall-bar shape. ‘Pt’ is the platinum electrode deposited on graphene, ‘CNT’ is the CNT carpet electrode grown on graphene, ‘G’ is the bare graphene electrode. ( b ) Three experiments that were used to measure the I–V responses: I, one probe contacts the platinum electrode and the other probe on the graphene electrode; II, one probe is on the platinum electrode, the other probe is suspended above the surface; III, one probe is on the platinum electrode, the other probe is contacting the CNT carpet side walls. ( c – e ) Characterization of a supercapacitor made from the graphene and CNT carpet hybrid materials. ( c ) Cyclic voltammetry of supercapacitor device under different scan rates. ( d ) Galvonostatic discharge curves under different discharge currents. ( e ) Ragone chart of energy density versus power density; the voltage window is 4 V. Full size image In addition to the efficient electrical connection, the new material also exhibits a large SSA of 2,000–2,600 m 2 g −1 , depending on the sample batch. The Brunauer–Emmett–Teller (BET) surface area of one batch of material is shown in Supplementary Fig. S6 . This sample has a BET SSA of 2,285 m 2 g −1 . The SSA of the graphene/CNT carpet hybrid material is comparable to the best reported values for open-ended CNTs (SSA 2,200 m 2 g −1 ) [28] and graphene/graphene oxide (SSA 2,000~3000, m 2 g −1 ) [29] . Considering the theoretical SSA limits of SWCNTs (1,315 m 2 g −1 for closed tubes, 2,630 m 2 g −1 for open-ended tubes) and graphene (2,630 m 2 g −1 ) [11] , the new material is attractive, as it has an SSA close to the limits without sacrificing electrical properties. Supercapacitors based on this graphene/CNT hybrid material were fabricated and the performance of the devices was tested. The results are shown in Fig. 3c–e . Additional information of device fabrication and more tested results are shown in the Supplementary Methods and Supplementary Fig. S7–S10 . The supercapacitor devices work properly up to 4 V and the energy density reaches a value >60 Wh kg −1 , which is among the highest reported values for all carbon-based supercapacitors. The growth metal substrates are directly used as the current collector for the supercapacitor; this design can potentially decrease the total weight of the final device. The life times of the devices were tested and no retention of the energy density was observed after 5,000 cycles ( Supplementary Fig. S10 ). The high performance of the device here is based upon a far simpler fabrication design ( Supplementary Fig. S7 ) than that used in most other similarly performing devices [29] , [30] . The results obtained beyond 2.7 V are formally outside the window of an electric double-layer capacitor and they extend into a region where redox activity may occur. However, the higher voltage measurements demonstrate the efficacy relative to the optimal performing supercapacitors to date [29] , [30] . Under the fabrication conditions in this work, the active surface area of electrode materials in the supercapacitor is estimated to be 517 m 2 g −1 ( Supplementary Methods ). The performance can be attributed to the high active surface area and the electrically connected material. A covalently bonded graphene–CNT junction No previous studies of the supposed nanotube–graphene junctions showed an atomic resolution junction between the two carbon materials. To understand how the CNTs connected to the graphene layer, an aberration-corrected STEM was used to investigate the atomic structure of the graphene–CNT junctions. A solvent-induced bundling effect was used to prepare the sample to directly observe the junction ( Supplementary Methods and Supplementary Fig. S12 ). 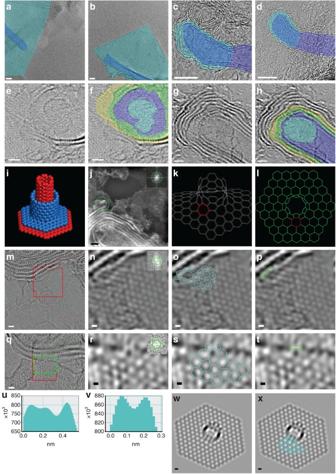Figure 4: TEM and STEM images of CNT–graphene junctions. (a,b) TEM images of the samples prepared by a solvent induce bundling method (Supplementary Fig. S12). The connection regions (roots) are directly observable. The cyan colour represents graphene planes and the blue colour represents the CNTs. (c,d) BF STEM images (band pass-filtered) of the CNT root regions. The blue colour represents CNTs and the cyan colour represents the additional shells on the root. Shown is a triple-walled nanotube incand a double-walled nanotube ind. Scale bar ina–d, 5 nm. (e–h) High-resolution BF STEM images of the root of CNTs;eandgare original STEM images (band pass-filtered);fandhare colour-enhanced images. The cyan colour represents the open-end region. The blue colour, green colour and yellow colour represent the nanotube walls. (i) The proposed model of the graphene and CNT junction. The CNT is covalently bonded to the graphene plane with additional shells (shown in blue) at the root. Scale bar ine–h, 1 nm. (j) ADF STEM image of the CNT–graphene junction. The image was filtered with band pass filter as indicated in the inset in the upper right corner. Scale bar inj, 1 nm. (k,l) Theoretical models suggested the atomic structure of the CNT–graphene junction12,13,14. Perspective view (k) and top-projected view (l). (m–t) High-resolution BF STEM images of CNT–graphene junctions. Scale bar inmandq, 0.5 nm. Scale bar inn–p, 0.2 nm. Scale bar inr–t, 0.1 nm. (m,q) The raw BF STEM images. (n,r) The high-resolution images after applying a filter (upper right inset) to the FFT of raw BF STEM images in the selected area (indicated as squares inmandq)31;nis from the red rectangle area inm;ris from the green rectangle area inq. (o,s) BF STEM images of junction areas with an overlayed structural sketch. (p,t) BF STEM images of junction areas with indicated areas for intensity profiles measurements. (u,v) Intensity profiles of indicated areas inpandt, respectively. (w) Simulated STEM image of CNT and graphene junction areas. Scale bar inw, 0.2 nm. (x) Simulated STEM image of CNT and graphene junction areas with an overlayed structural sketch. Scale bar inx, 0.2 nm. Figure 4a are conventional TEM images (taken at 200 KV) of the CNT root regions where they connect to the graphene plane. Figure 4c are the bright field (BF) STEM images (at 80 KV) of the roots of two CNTs. Interestingly, although the CNTs are few-walled tubes (triple-walled CNT Fig. 4c , double-walled CNT Fig. 4d ), additional shells are often found at the roots (additional images are shown in Supplementary Fig. S16 ). The additional shells may produce a stronger CNT root that could in turn benefit the alumna lift process. In Fig. 4e–h , the lateral layers inside the CNT (indicated by the cyan colour in Fig. 4f ) are observed, which implies that the CNTs are open-ended at the bottom. This agrees with theoretical prediction [12] , [13] , [14] that the CNT should be open-ended when it forms covalent bonds with the graphene base layer. The innermost rings of the indicated area (cyan colour) in Fig. 4f still have visible graphitic structure because of the upper walls of the CNT. The BET SSA results reported above also suggest that the CNTs are open-ended. The simulated STEM images and additional experimental STEM images ( Supplementary Fig. S14 ) confirmed that a ring-like structure is a characteristic property for covalent bonds between CNTs and graphene, and has not been observed in prior work. On the basis of those observations, a possible model of the CNT–graphene junction is proposed in Fig. 4i . The CNT is covalently bonded to the graphene plane and additional shells are formed in the CNT root region. This model implies that the outermost shell of the nanotube root will be bonded to the topmost layer of graphene, which was also directly observed in the annular dark field (ADF) image in Fig. 4j . As in Fig. 4j , the left green circled area shows that a scrolled graphene layer and the outermost shell of the CNT are the same layer. Previous theoretical work [12] , [13] , [14] suggested the detailed atomic structure of the CNT and planar graphene transformations, which are shown in Fig. 4k . A characteristic property of the junction is the existence of seven-member rings on the bonding region (indicated in red in Fig. 4k ). From the projection drawing ( Fig. 4l ), the lower four benzene rings connected to the seven-membered ring should be mostly planar, and the upper three rings are more distorted. Fig. 4m–t show observed atomic structure of two junction regions. In the enlarged images ( Fig. 4n–p ), each white spot represent an aromatic ring. The number of edges for each ring can be identified by counting the adjacent white spots. As in Fig. 4o , the seven-member rings correspond to the junction region as shown in the structure drawing. Their positions, with four rings in the graphene plane and three rings distorted because of their out-of-plane orientations, match the simulation results ( Figs 4k ). The intensity profiles ( Fig. 4p ) are used to identify those close aromatic rings. The simulated BF STEM images of CNT–graphene junctions based on structures proposed by the theoretical papers [12] , [13] , [14] , ( Supplementary Figs. S13 and S15 ) are presented in Fig. 4w , which well-match the observed BF STEM images ( Supplementary Fig. S15 ). Taken together, the STEM images confirm the existence of covalent bonds between the CNTs and graphene in junction areas. This result is consistent with the conjugated seven-membered-ring-containing junctions suggested by theoretical studies. This structure further explains the high SSA and ohmic connections that were observed. Figure 4: TEM and STEM images of CNT–graphene junctions. ( a , b ) TEM images of the samples prepared by a solvent induce bundling method ( Supplementary Fig. S12 ). The connection regions (roots) are directly observable. The cyan colour represents graphene planes and the blue colour represents the CNTs. ( c , d ) BF STEM images (band pass-filtered) of the CNT root regions. The blue colour represents CNTs and the cyan colour represents the additional shells on the root. Shown is a triple-walled nanotube in c and a double-walled nanotube in d . Scale bar in a – d , 5 nm. ( e – h ) High-resolution BF STEM images of the root of CNTs; e and g are original STEM images (band pass-filtered); f and h are colour-enhanced images. The cyan colour represents the open-end region. The blue colour, green colour and yellow colour represent the nanotube walls. ( i ) The proposed model of the graphene and CNT junction. The CNT is covalently bonded to the graphene plane with additional shells (shown in blue) at the root. Scale bar in e – h , 1 nm. ( j ) ADF STEM image of the CNT–graphene junction. The image was filtered with band pass filter as indicated in the inset in the upper right corner. Scale bar in j , 1 nm. ( k , l ) Theoretical models suggested the atomic structure of the CNT–graphene junction [12] , [13] , [14] . Perspective view ( k ) and top-projected view ( l ). ( m – t ) High-resolution BF STEM images of CNT–graphene junctions. Scale bar in m and q , 0.5 nm. Scale bar in n – p , 0.2 nm. Scale bar in r – t , 0.1 nm. ( m , q ) The raw BF STEM images. ( n , r ) The high-resolution images after applying a filter (upper right inset) to the FFT of raw BF STEM images in the selected area (indicated as squares in m and q ) [31] ; n is from the red rectangle area in m ; r is from the green rectangle area in q . ( o , s ) BF STEM images of junction areas with an overlayed structural sketch. ( p , t ) BF STEM images of junction areas with indicated areas for intensity profiles measurements. ( u , v ) Intensity profiles of indicated areas in p and t , respectively. ( w ) Simulated STEM image of CNT and graphene junction areas. Scale bar in w , 0.2 nm. ( x ) Simulated STEM image of CNT and graphene junction areas with an overlayed structural sketch. Scale bar in x , 0.2 nm. Full size image In all previously reported experimental work [21] , [22] , [23] , [24] on similar three-dimensional graphene and CNT hybrid materials, the high-quality, single- and few-walled CNT carpets were not grown, nor were they shown with demonstrated seamless junction. To introduce the direct contact between a graphitic substrate and the CNTs, there was typically no buffer layer, which results in low surface area, multi-walled CNT growth. The key step in this work is to introduce the floating buffer layer. The direct Odako tip growth of the CNT carpet on the graphene substrate was promoted when the catalyst could be raised with the buffer layer, resulting in covalent bonding between the graphene substrate and the CNT roots. If that catalysts remains at the surface, consumption of the graphene will ensue, as the graphene will be used as a nanotube carbon growth source. In conclusion, we disclosed a method to build and microscopically confirm covalent bonds between graphene and CNT carpets. The aberration-corrected STEM revealed the atomic structure of conjugated covalent bonds in the junction region, which is in agreement with previous simulation studies. Without sacrificing their stand-alone properties, the ohmic interconnected graphene and CNT carpet hybrid can be produced in a high-surface area material that can affect, for example, high-performance supercapacitor devices. These findings broaden our understandings of the graphene–CNT materials union and may lead to advances in areas such as energy storage and electronic devices. Graphene and CNT carpet hybrid material synthesis The graphene is grown on copper foil (25 μm thick) using reported methods [17] , [18] , [20] . The catalyst (1 nm iron) and buffer layer (3 nm Al 2 O 3 ) were deposited in series on the graphene-covered copper foil by e-beam evaporation. The growth of the CNT carpet can be done at either atmospheric or reduced pressure. When the experiment was done at atmospheric pressure, the flow rates of ethylene, hydrogen and argon were 100, 400 and 500 sccm, respectively. A bypass channel was used to bubble water vapour into the system and hydrogen was used as the carrier gas. The flow rate for the bubbling hydrogen is 10 sccm. Before starting the carbon-source flow, the assembled sample was annealed in the furnace under the same environment, except the carbon source was closed. The annealing was performed at 750 °C for 3 min. After annealing, the carbon source was introduced and the growth time depended on the carpet growth height that was sought. Typically, a 10-min growth will yield a carpet with a height of ~120 μm. When the experiment was done at reduced pressure, a water-assisted hot filament furnace was used [25] . The flow rate of acetylene and hydrogen were 2 and 210 sccm, respectively. The flow rate for the bubbling hydrogen was 200 sccm. The sample was first annealed at 25 Torr for 30 s, during which a tungsten filament was activated by tuning the working current to 9–10 A and a power of 45 W to reduce the catalyst. Then, the pressure was reduced to ~5 Torr and the hot filament was switched off immediately to start the nanotube growth for additional 1–10 min, depending on the carpet height sought. Typically, a 10-min growth period will yield carpet with a height of ~60 μm. Characterization methods SEM images were taken using a JEOL6500 SEM and a FEI Quanta 400-field emission gun SEM. TEM images were taken using a 200-kV JEOL FE2100 TEM. Atomic resolution STEM images were collected with a JEOL JEM-ARM200F operated at 80 kV equipped with a Cs probe corrector. Collection angles for the ADF images were set to 33 and 125 mrad for the inner and outer semi-angles. For the BF images, the collection angle was 7.5 mrad. The convergence angle was set to 24 mrad. Dwell pixel time was set at 64 μs. Aberrations up to third order were corrected through a dodecapole corrector aligned through the CESCOR software. After the samples were transferred to the STEM chamber, they were beam-showered for 10 min to decrease the charging effect. The BET experiment was done using a Quantachrome Autosorb-3B surface analyser, and the sample was dried at 110 °C under vacuum for 16 h before the experiment. The Raman spectra of the samples were recorded with a Renishaw Raman RE01 scope using a 633- and a 514-nm argon laser. How to cite this article: Zhu Y. et al . A seamless three-dimensional carbon nanotube graphene hybrid material. Nat. Commun. 3:1225 doi: 10.1038/2234 (2012).